Enhanced Moran effect by spatial variation in environmental autocorrelation Spatial correlations in environmental stochasticity can synchronize populations over wide areas, a phenomenon known as the Moran effect. The Moran effect has been confirmed in field, laboratory and theoretical investigations. Little is known, however, about the Moran effect in a common ecological case, when environmental variation is temporally autocorrelated and this autocorrelation varies spatially. Here we perform chemostat experiments to investigate the temporal response of independent phytoplankton populations to autocorrelated stochastic forcing. In contrast to naive expectation, two populations without direct coupling can be more strongly correlated than their environmental forcing (enhanced Moran effect), if the stochastic variations differ in their autocorrelation. Our experimental findings are in agreement with numerical simulations and analytical calculations. The enhanced Moran effect is robust to changes in population dynamics, noise spectra and different measures of correlation—suggesting that noise-induced synchrony may play a larger role for population dynamics than previously thought. Understanding the causes and mechanisms underlying spatial synchrony of biological populations has become a key issue in population ecology [1] , [2] , [3] , [4] , [5] , [6] . Several mechanisms for explaining population synchrony have been put forward, such as dispersal between populations and spatially extended trophic interactions [6] . Synchrony may also arise from spatially correlated environmental influences (Moran effect [7] , [8] ). Moran (1953) suggested that spatially separated populations, which are regulated by the same density-dependent structure, will tend to fluctuate in synchrony if they are exposed to similar environmental variation. In particular, in the special case of linear density dependence the cross-correlation between the regional populations, r p , will be identical to that of the environment, r p = r . This statement became known as Moran theorem [7] . Given that environmental fluctuations can be spatially correlated over large distances, the Moran effect was considered as a major mechanism for generating population synchrony under natural [9] , [10] , [11] , [12] , [13] , [14] and laboratory conditions [15] , [16] , [17] . It was generalized to include nonlinear density dependence, populations in nonidentical habitats, the influence of dispersal, cyclic populations, species interactions and various combinations of these factors [9] , [12] , [18] , [19] , [20] , [21] , [22] , [23] . All these studies found that the correlation of independent populations, not coupled by dispersal, remains bounded by the environmental correlation, r p ≤ r , which should limit the Moran effect as a driver of population synchrony. Here we show that the magnitude of the Moran effect can be substantially enhanced, r p > r , in the common ecological case that the environmental fluctuations are temporally autocorrelated and this autocorrelation varies spatially. Temporal autocorrelation refers to a relationship between successive observations in a time series and can be described by its noise colour. The term ‘colour’ derives from the analogy between the spectral representation of Fourier-transformed time series and the spectrum of (visible) light. A noisy signal is called ‘white’ if successive values are uncorrelated so that no frequency dominates. In contrast, red noise indicates positive autocorrelation, that is, successive values are more similar than expected by chance. Time series with red noise are dominated by low-frequency fluctuations and are often found in nature, for example, in climate variables and population densities [24] , [25] , [26] , [27] , [28] , [29] . The colour of environmental noise can have a substantial influence on population dynamics and persistence [26] , [30] , [31] , [32] , [33] , [34] , [35] but, although relevant, its effect on population synchrony has rarely been addressed. Previous theoretical investigations revealed that reddened environmental noise may intensify spatial synchrony [19] , [30] , [36] , [37] , [38] . These investigations, however, were restricted to the case of identical noise colours in all populations, despite the fact that empirical studies of a wide range of environmental variables have revealed substantial variations in noise colour between geographic regions and on gradients from land to the ocean [24] , [26] , [29] , [39] , [40] , [41] . In this communication, we study the Moran effect in response to spatial variations in habitat properties and environmental autocorrelation (noise colour). While spatial variability is commonly thought to reduce population synchrony [12] , [19] , [20] , [23] , here we perform a series of laboratory experiments to show that it may either suppress or enhance the intensity of noise-induced spatial synchronization: (i) in the absence of spatial variations (identical habitats and noise colours) we reproduce the Moran theorem, r p = r ; (ii) spatial variations in habitat properties suppress the Moran effect, r p < r ; and (iii) we provide evidence from experiments, theoretical analyses and numerical simulations that the Moran effect can be significantly enhanced, r p > r , by spatial variations in environmental autocorrelation. Thus, our major finding is the counterintuitive result that the correlation between otherwise independent populations can be larger than that of their respective environments (enhanced Moran effect) if the populations experience environmental fluctuations with different noise colour. We demonstrate this effect in experiments with living organisms under well-defined conditions, using chemostats containing populations of the green alga Chlorella vulgaris (Chlorococcales). We investigate the population dynamics of two isolated populations, N A and N B , experiencing correlated environmental stochasticity ( Fig. 1 ). We impose environmental variation on the chemostat populations by altering the dilution rates, δ A ( t ) and δ B ( t ), at discrete time intervals of 1 or 2 h, using computer-generated random numbers. Thereby, the dilution rates are cross-correlated by r = C ( δ A , δ B ) and autocorrelated with noise colours α and β . This stochastically correlated forcing is the only way in which the two systems are coupled. Using light extinction as a proxy of algal biomass [42] , we measure the population densities with an unusually high temporal resolution of 5-min intervals. The two populations respond to the stochastic forcing with fluctuations that are cross-correlated by r p = C ( N A , N B ). This population correlation, in general, is different to the correlation of the input signals. Thus, this experimental set-up allows us to model environmental variation and its synchrony, as well as the population response and transformation of this synchrony (that is, the Moran effect) in a well-controlled laboratory system. 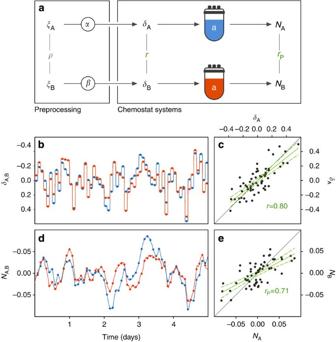Figure 1: Noise-induced synchronization in two independent populations. (a) Experimental set-up to explore the response of two populationsNAandNBto correlated stochastic forcing, realized as chemostat systems ofC. vulgaris. The two systems are coupled only by their correlated noise input, which is generated by data preprocessing. For each system, Gaussian distributed white noises,ξA(t) andξB(t), are generated that are cross-correlated byρ=C(ξA,ξB). To implement temporal structure, the generating noises are filtered through an autoregressive AR(1) process with autocorrelation parametersαandβ, respectively. The resulting time series determine the experimental dilution rates (δA(t),δB(t)) of the chemostats in defined time intervals Δtand are cross-correlated byr=C(δA,δB). The correlation between chemostat population densitiesNA(t) andNB(t) is then measured byrp=C(NA,NB). (b–e) Typical population response (here shown for the case of two identical populations and white noise,α=β=0, trial 1). (b) Normalized dilution ratesδA(t) andδB(t) andd, normalized population densitiesNA(t) andNB(t) of system A (blue) and system B (red). Circles indicate the respective values at the time instances when dilution rates were set to a new value. Further shown is the pairwise correlation (black circles) and the regression line (green) of normalized dilution ratesr=0.80 (c) and of population densitiesrp=0.71 (e). The green dotted lines show the 95% confidence intervals; 0.68≤r≤0.87 (s.e.=0.047) and 0.56≤rp≤0.82 (s.e.=0.064). For illustration, the diagonal is indicated as black line. Figure 1: Noise-induced synchronization in two independent populations. ( a ) Experimental set-up to explore the response of two populations N A and N B to correlated stochastic forcing, realized as chemostat systems of C. vulgaris . The two systems are coupled only by their correlated noise input, which is generated by data preprocessing. For each system, Gaussian distributed white noises, ξ A ( t ) and ξ B ( t ), are generated that are cross-correlated by ρ = C ( ξ A , ξ B ). To implement temporal structure, the generating noises are filtered through an autoregressive AR(1) process with autocorrelation parameters α and β , respectively. The resulting time series determine the experimental dilution rates ( δ A ( t ), δ B ( t )) of the chemostats in defined time intervals Δ t and are cross-correlated by r = C ( δ A , δ B ). The correlation between chemostat population densities N A ( t ) and N B ( t ) is then measured by r p = C ( N A , N B ). ( b – e ) Typical population response (here shown for the case of two identical populations and white noise, α = β =0, trial 1). ( b ) Normalized dilution rates δ A ( t ) and δ B ( t ) and d , normalized population densities N A ( t ) and N B ( t ) of system A (blue) and system B (red). Circles indicate the respective values at the time instances when dilution rates were set to a new value. Further shown is the pairwise correlation (black circles) and the regression line (green) of normalized dilution rates r =0.80 ( c ) and of population densities r p =0.71 ( e ). The green dotted lines show the 95% confidence intervals; 0.68≤ r ≤0.87 (s.e.=0.047) and 0.56≤ r p ≤0.82 (s.e.=0.064). For illustration, the diagonal is indicated as black line. Full size image Identical chemostat systems We present results from three different experimental scenarios. First, we tested whether populations would follow the behaviour expected from the Moran theorem. For this, we parameterized both chemostat systems identically, imitating identical habitats, that is, the average dilution rates and the resource supply concentrations had the same value for both systems (see Methods). In six consecutive runs, the populations experienced white noise ( α = β =0) that was cross-correlated between the two populations with coefficients r in the range from 0 to 1 (for parameters and exact values of r see Table 1 ). The populations responded to the stochastic forcing with correlated population dynamics, with cross-correlations that correspond to that of the environmental forcing, r p ≈ r (see Fig. 2a ). These results agree with the prediction from the Moran theorem and confirm the hypothesis that correlated stochastic forcing can synchronize the dynamics of noninteracting populations. Table 1 System characteristics of all experimental trials. 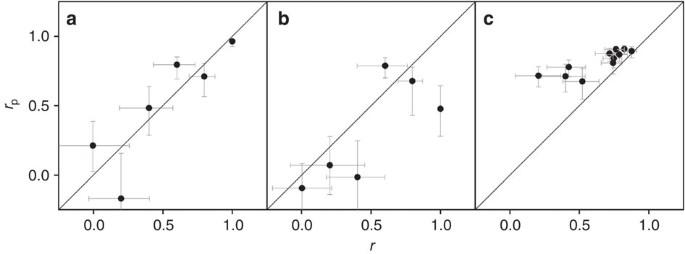Figure 2: Moran effect in different experimental treatments. Population correlationrpin dependence of the environmental correlationr(black circles). (a) Identical systems, white noise: the correlation of the population equals that of the environmentrp=r(Moran theorem). (b) Non-identical systems, white noise: the population correlation is smaller than the environmental correlationrp≤r. (c) Identical systems, differently autocorrelated noise. Even though the two populations are non-interacting, the correlation of the populations exceeds that of the environmentrp>r(enhanced Moran effect). Error bars show 95% confidence intervals from a sample of 10,000 noise replicates (r), and from resampling measured correlations by bootstrapping (rp). The diagonal lines indicate the expected outcome of the Moran theoremrp=r. Full size table Figure 2: Moran effect in different experimental treatments. Population correlation r p in dependence of the environmental correlation r (black circles). ( a ) Identical systems, white noise: the correlation of the population equals that of the environment r p = r (Moran theorem). ( b ) Non-identical systems, white noise: the population correlation is smaller than the environmental correlation r p ≤ r . ( c ) Identical systems, differently autocorrelated noise. Even though the two populations are non-interacting, the correlation of the populations exceeds that of the environment r p > r (enhanced Moran effect). Error bars show 95% confidence intervals from a sample of 10,000 noise replicates ( r ), and from resampling measured correlations by bootstrapping ( r p ). The diagonal lines indicate the expected outcome of the Moran theorem r p = r . Full size image Variation in habitat properties Second, we tested whether stochastic forcing is able to synchronize populations that differ in their key habitat properties. For this, we imposed different values of average turn-over rate (dilution) and carrying capacity (resource supply concentrations) on the two systems, so that one habitat was characterized by high nutrient availability but also high mortality, whereas both factors were lower in the other one (see Methods). Again, the populations experienced six treatments of white noise with cross-correlation coefficients in the range between 0 and 1 (for exact values and parameters see Table 1 ). In our experiments we observed that stochastic forcing is able to synchronize even populations living in non-identical habitats ( Fig. 2b ). However, the cross-correlation of population density was consistently smaller than that of the environmental driving, r p < r . This finding confirms results from field and theoretical studies [12] , [19] , [20] , [23] . Variation in environmental autocorrelation In the third scenario, we tested the response of two populations with identical habitats under the influence of differently autocorrelated noise. In theory (see Methods) this would allow for enhancing input noise correlations, r p / r >1. For this, the two experimental populations were adjusted to have identical habitat conditions. However, in contrast to the previous scenarios, we implemented temporal autocorrelations (noise colour) in the time series of dilution rates (see Methods). We performed a series of 11 experimental runs, each representing a combination of differing autocorrelation parameters α and β roughly adjusted within the range [0,0.9] (see Table 1 ). In our experiments we observed that in autocorrelated environments the correlation of the populations can significantly exceed that of the environmental shocks ( Fig. 2c ). To compare this experimental finding with theoretical expectations, we plot the synchrony amplification factor r p / r as a function of the realized noise correlation r and the difference in autocorrelation parameters | α − β | ( Fig. 3 ). A value of r p / r =1 (solid line in Fig. 3 ) corresponds to the expectation from the Moran theorem. However, the experimental findings demonstrate that, in contrast to the naive expectation, the input correlation of the environmental fluctuations is amplified by the population dynamics, by more than 300% for large differences in autocorrelation parameters. This synchrony amplification, r p / r , increases in strength as the difference in noise colours | α − β | becomes more pronounced. 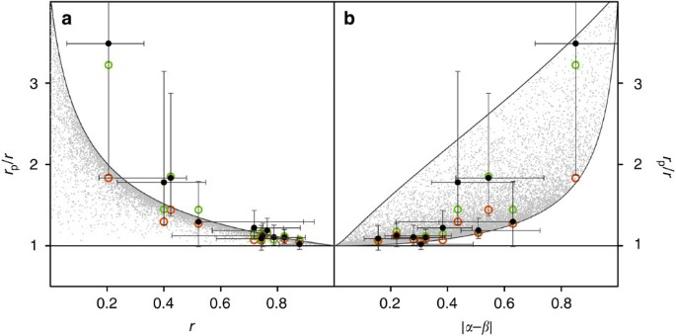Figure 3: Enhanced Moran effect in differently autocorrelated environments. Observed correlation amplification factorrp/r(black filled circles) as a function of (a) the environmental correlationr(α,β) and (b) the difference in autocorrelation parameters |α−β|. Red circles show the amplification factors theoretically expected from an AR(1)-process witha=0.97 (equation 7) for the respective, experimentally realized parameter combinationr(α,β); green circles show the amplification factors obtained from chemostat simulations (equation 11). Grey dots show amplification factors simulated by an AR(1)-process for 20,000 randomly chosen autocorrelation parametersαandβ, taken from a uniform distribution in the range [0,1]; grey lines give the upper and lower boundaries. Error bars show 95% confidence intervals from a sample of 10,000 noise replicates (rand |α−β|), and from resampling measured correlations by bootstrapping (rp/r). The horizontal linesrp/r=1 indicate the expected outcome according to the Moran theorem. Figure 3: Enhanced Moran effect in differently autocorrelated environments. Observed correlation amplification factor r p / r (black filled circles) as a function of ( a ) the environmental correlation r ( α , β ) and ( b ) the difference in autocorrelation parameters | α − β |. Red circles show the amplification factors theoretically expected from an AR(1)-process with a =0.97 (equation 7) for the respective, experimentally realized parameter combination r ( α , β ); green circles show the amplification factors obtained from chemostat simulations (equation 11). Grey dots show amplification factors simulated by an AR(1)-process for 20,000 randomly chosen autocorrelation parameters α and β , taken from a uniform distribution in the range [0,1]; grey lines give the upper and lower boundaries. Error bars show 95% confidence intervals from a sample of 10,000 noise replicates ( r and | α − β |), and from resampling measured correlations by bootstrapping ( r p / r ). The horizontal lines r p / r =1 indicate the expected outcome according to the Moran theorem. Full size image Theoretical analysis The phenomenon of an enhanced Moran effect is confirmed by theoretical analysis. Linear theory allows the amplification factor r p / r to be calculated for independent populations, having identical linear population demography described by the density regulation parameter a (see Methods, equation 7). Expanding this result for small values of a and differences in autocorrelation | β − α | yields The deviation between the synchrony amplification factor and the expectation from the Moran theorem, r p / r −1, scales quadratically with both the difference in autocorrelation, α − β , and the density regulation parameter a . Thus, in independent populations described by linear demography the cross-correlation of population numbers can be larger than that of their stochastic environment, r p ≥ r . Such an enhanced Moran effect arises if the noise colour differs between the two populations, | β − α |>0. If both autocorrelation parameters are equal, α = β , the Moran theorem r p = r is reproduced. Note that it is not the noise colour in itself, but its variation between habitats, which is crucial for an enhanced Moran effect. In fact, with increasing autocorrelation parameters in both populations, their difference | β − α | must eventually obtain a small value, which inhibits synchrony amplification. This conforms to classic findings about the tracking error to environmental variability [32] . More reddened noise in both systems should enable the populations to track the environment more closely, thereby reducing the possibility of an enhanced Moran effect. These analytic results are confirmed by the experimental findings ( Fig. 3 ). Interestingly, in general, the experiments showed even larger values of the amplification factor r p / r than predicted from linear theory. Numerical simulations with time-continuous chemostat models, closely following the experimental system (see Methods and Supplementary Fig. 2 ), were in agreement with the experimental findings and showed that these results are robust. We could observe the enhanced Moran effect in very different settings. It prevailed for different measures of cross-correlation ( Supplementary Fig. 6 ), for higher-order autoregressive population dynamics ( Supplementary Figs 10 and 11 ), for non-identical populations, that is, when the population regulation parameter a varied between two populations ( Supplementary Fig. 12 ), and nonlinear population dynamics (realized as two noise-driven logistic maps, Supplementary Fig. 13 ). These simulations confirm that non-identical or nonlinear population dynamics, in general, suppress noise-induced synchrony, but show also that the enhanced Moran effect is maintained even under these conditions. Finally, correlation amplification also prevailed for different types of autocorrelated noise, including 1/ f β -noise ( Supplementary Fig. 14 ). Our simulations show that the correlation amplification factor increases with the difference in spectral exponents also for long-term correlations in the noise; however, the dependence on the noise colour can be non-monotonous so that the largest correlation amplification is obtained for intermediate values of noise colour. How can this counterintuitive behaviour be explained? On the basis of fundamental information theoretic concepts, the mutual information between two non-interacting systems (a measure of the full statistical interdependence) cannot increase. Thus, the mutual information between the population densities { N A ( t ), N B ( t )} cannot exceed the mutual information between the driving signals { δ A ( t ), δ B ( t )}. However, this does not apply to the (Pearson) cross-correlation coefficient, which evaluates the signal values in both systems at the same time instances, while the full temporal history in the mutual relationship between two signals is coded in the cross-correlation function, or equivalently the cross-spectrum [7] , [43] . If two autocorrelated signals differ in their noise colour, α ≠ β , some mutual interdependence, that is inherently present in the signals, will be distributed differently in the frequency components and can, in principle, not be detected by means of the cross-correlation coefficient. In our experimental setting this is evident in the reduced correlation r of the autocorrelated dilution rates compared with the larger correlation ρ of the white generating noises ( Fig. 1a ). This hidden correlation in the stochastic driving signals can be unmasked, when it is imposed on a population that effectively responds to the stochastic forcing as a low-pass filter (see Methods). Thereby, increasing the difference in autocorrelation, α − β , does not result in an enhanced population synchrony. Instead, larger differences in noise colour reduce the correlation r between the environmental variables more strongly than the correlation r p between the population densities. As a consequence, the ratio between input and population signals, that is, the correlation amplification factor r p / r , can increase—which finally leads to the enhanced Moran effect. From the perspective of a ‘super-observer’, with full information also about the generating time series ξ A,B ( t ), this effect may not seem to be very surprising. An omniscient observer, however, does not reflect ecological reality. In the field, an observer will experience only the environmental signals acting on the populations (together with their corresponding auto- and cross-correlation), without information about the underlying causes that have generated these time series. From the perspective of this field observer, the measurable input noise correlation is ‘surprisingly’ enhanced when it is passed through the AR-filter of the non-interacting populations. These problems can be resolved by taking the full mutual relationship between multivariate signals into account. Notwithstanding this, it is the common praxis in ecological field studies to quantify population synchrony by the cross-correlation coefficient, even though it yields a restricted insight into the time series. Our findings are thus highly relevant for the understanding of field observations where differently autocorrelated time series prevail. In our experimental exploration of the enhanced Moran effect, we covered the wide range of spatial variation in autocorrelation that is known from empirical studies of environmental variables, including air and water temperatures in and around lakes, rivers and oceans [24] , [26] , [29] , [39] , [40] , [41] . Organisms distributed over broad ranges or even on a global scale are very likely to be encountered in such habitats. This is especially true for eukaryotic microorganisms [44] and many phyto- and zooplankton species [45] , [46] often possessing the key roles in their habitats. On the basis of these observations, we should expect differently autocorrelated environmental variability, as used in our experiments, to be prominent in wild populations. On the other hand, in the field not all implicit assumptions that went into the design of our model set-up will be completely satisfied. In free-living populations, the Moran effect will be further complicated by additional confounding factors, such as differences in habitat properties, density dependence, trophic interactions, long-range dispersal or long-term correlations. All these factors can potentially interfere with the intensity of noise-induced population synchrony, which sets limitations to the applicability of our analytic formulaequations (1) and (7). Our numerical simulations revealed, however, that the phenomenon of an enhanced Moran effect is robust to such factors, confirming that our main results also hold under more general settings, at least qualitatively (see Supplementary Figs 10–14 ). The derivation of our main theoretical result, equations (1) and (7), is not specific to ecological populations and should apply in general to linear systems under the influence of differently autocorrelated noise. Thus, the enhancement of the Moran effect by spatial variation in autocorrelation is universal and should play an important role also in other disciplines where autocorrelated stochastic influence is prominent. Important examples are the synchronization of epidemic outbreaks (for example, Cholera [47] or Malaria [48] ) in separate regions by climate events, the functioning and correlated firing in populations of neurons in different regions of the cortex [49] , [50] , and the regulation of genetic and biochemical networks [51] , [52] . Chemostat set-up Monoclonal batch cultures of the green algae C. vulgaris (Chlorococcales) were kept in a climate chamber at 23.3±0.4 °C and constant fluorescent illumination at 110 μE m −2 s −1 (preventing synchronization by light–dark cycles) and served as stock cultures for the chemostat experiments. Resource concentrations were adjusted to be nonlimiting or only weakly limiting (nitrogen being the growth-limiting resource). We used sterile, modified Woodshole WC medium after Guillard & Lorenzen (1972, pH=6.8). Nitrogen concentrations were sufficiently low to limit algal growth and were set to 80 μmol l −1 (phosphorus to nitrogen ratio P / N 80 =1/1.6) by adjusting the amount of NaNO 3 . The medium contained trace metals, vitamins and other nutrients in non-limiting concentrations. For stock cultures we used medium containing a nitrogen concentration of 320 μmol l −1 . We used glass chemostat vessels of 1.5 l volume and adjusted the culture volume to ~800 ml. To provide homogeneous mixing and to prevent CO 2 limitation, algal cultures were bubbled with pressurized, sterile air. We used an automated light extinction measurement system [42] , [53] , [54] . Light extinction was measured as light transmittance (wavelength=880 nm) through a sterile syringe that pulled out and pushed back 10 ml of chemostat content every 5 min, being therefore a quasi-continuous, noninvasive method. Experimental procedure When the phytoplankton populations had reached a steady state, we imposed correlated environmental variability on the chemostats for a duration of 5 days. For this, we automatically altered the dilution rates at discrete time intervals Δ t , using computer-generated random numbers to steer the peristaltic pumps (see Supplementary Fig. 1 for an exemplary illustration of the influence of the dilution rate on population densities and growth rates). Thereby, the pairwise cross-correlation and the temporal autocorrelation of the sequence of dilution rates were adjusted to a pre-determined value. The communication between the computer and the peristaltic pumps was realized by digital/analog input/output converters (Texas Instruments). The experiments comprise three scenarios. In the first scenario (see Fig. 1 ), we set up two ( N =2) identical chemostat systems, parameterized by average dilution rate, ‹ δ A ›=‹ δ B ›=0.75 per day, and resource (nitrogen) supply concentration, R i,A = R i,B =80 μmol l −1 . In six consecutive runs, the populations experienced white Gaussian noise with s.d. σ =0.2 that was cross-correlated between the two populations with coefficients r of ~0.8, 0.2, 0.6, 0.0, 0.4 and 1.0 (for exact values see Table 1 ). Subsequent values of correlation coefficients were chosen not to be in ascending or descending order to avoid systematic errors. The s.d. was small enough to avoid the occurrence of negative values in the noise generation process. The length of the time interval between dilution rate changes was Δ t =2 hours, which allowed a total number of n =60 random shocks. Both, s.d. and interval length of the stochastic forcing ensured significant effects on the populations. In the second scenario, we set up two chemostats with differing levels of dilution rates, ‹ δ A ›=0.75 per day, ‹ δ B ›=0.40 per day, and resource supply, R i,A =80 μmol l −1 , R i,B =40 μmol l −1 (see Table 1 ). Again, the populations experienced six treatments of white noise that was cross-correlated in the range from 0 to 1 as in scenario 1 with Δ t =2 h. Given the lower value of ‹ δ B ›, the s.d. was decreased to σ =0.15 to make the occurrence of negative values in the noise generation process of δ B unlikely. In the third scenario, we tested for synchrony in populations living in differently autocorrelated habitats. We used a set-up of up to N =4 chemostats, which allowed us to measure N ·( N −1)/2=6 independent pairwise correlations of population densities in a single experimental run (see below). Basic habitat properties were again identical (cf. first scenario); however, we decreased the interval length to Δ t =1 hour in order to double the number of data points ( n =120). This was necessary to improve the statistical significance in the autocorrelated environments where the random shocks are not independent. Simultaneously, we increased the s.d. of the dilution rates to σ =0.25 to ensure distinct responses in population densities (again avoiding negative values of dilution rates; Supplementary Figs 4 and 5 exemplify the influence of noise colour on population densities and growth rates). Data analysis Population synchrony between two time series x ( t ) and y ( t ) was measured as Pearson’s correlation coefficient Generation of autocorrelated noise We used a two-step data preprocessing to generate noises δ i ( t ) ( i =1… N ) that are pairwise cross-correlated with the desired correlation r ij and temporally autocorrelated with α i (that is, the noise colour). First, we generated cross-correlated, but not temporally correlated, ‘generating noises’. For this we used N independent white noises ζ i ( t ), taken from Gaussian distributions with zero mean and variance σ 2 =1. These independent noises were multiplied with a correlation matrix A to establish the N generating noises ξ i ( t ) that are pairwise correlated with adjustable parameters ρ ij = C ( ξ i ( t ), ξ j ( t )). Thus, ξ ( t )= Aζ ( t ) with the matrix ( N =4) with diagonal elements: , , , and off-diagonal elements a 21 = ρ 21 , a 31 = ρ 31 , a 41 = ρ 41 and a 32 =( ρ 32 −a 31 a 21 ) /a 22 , a 42 =( ρ 42 − a 21 a 41 ) /a 22 , a 43 =( ρ 43 − a 31 a 41 −a 32 a 42 )/ a 33 . For smaller values of N we used a submatrix of A (for example, to generate two time series, N =2, we used A =[1 0, a 21 a 22 ]). N ote that the generating noises were introduced for computational convenience and bear no ecological meaning. In the second step, we added temporal structure (that is, noise colour) into the ξ i ( t ), using a first-order autoregressive AR(1) process [32] , [43] with autocorrelation parameters α i (| α i |<1, parameters α and β in Fig. 1 ). Thereby, the pairwise correlations between the noises are reduced to [19] , [20] After scaling to the desired s.d. and adding the mean dilution rate, we finally obtained the actual environmental noises δ i ( t ) that are acting on the populations. As negatively autocorrelated (blue) noise is rare (or rather not present) in ecological systems, we chose most of the autocorrelation parameters α i to range within 0.0 and 0.9. The actually realized autocorrelation in the finite time series (measured by regression analysis and using the Matlab function ‘arcov’) slightly deviated from this value (see Table 1 ). In one experimental run (trial 19), we obtained an autocorrelation that was slightly negative (−0.18). In this procedure, the pairwise correlations ρ ij of the generating noises are free parameters. They can in principle be set to ρ ij =1, to achieve maximal pairwise correlations of the dilution rates. In reality, however, environmental signals will rarely be correlated by the maximal possible value that is consistent with their specific autocorrelation. Therefore, we used a different parametrization and in the experiment adjusted the ρ ij to a smaller value. For convenience, we used so that the pairwise correlations between the dilution rates are given as . Data processing Before computing the correlation coefficients, all population time series (from experiments and from simulations) underwent identical data processing ( Supplementary Fig. 3 ). First, the logarithmic light extinction values were normalized to zero mean. Second, the time series were smoothed by a local regression filter that uses weighted linear least squares and a second-degree polynomial model (‘rloess’ filter from Matlab’s curve fitting toolbox, the span was set to 2% of the data points). Third, we applied detrending by subtracting a coarse fit that was generated with a Savitzky–Golay filter. This filter comprises a generalized moving average with coefficients determined by an unweighted linear least-squares regression and a second-degree polynomial model (‘sgolay’ filter from Matlab’s curve fitting toolbox, the span was set to 100% of the data points). Finally, the resulting time series was stroboscopically sampled at regular time intervals Δ t corresponding to the alterations in the dilution rate δ ( t ), to obtain the discrete times series N ( t ) of the population densities. Analytic derivation of the enhanced Moran effect We use an AR(1) process to model the dynamics of two populations ( A and B ) at the discrete times t =1… n when the dilution rates are changed ( Fig. 1 ). Here N A ( t ), N B ( t ) describe the log-transformed population densities, the noise terms δ A ( t ), δ B ( t ) are generated as described above and the density regulation parameter | a |<1 so that the AR(1)-process is stationary [7] . Analysis of the experimental and simulated population densities showed that an AR(1)-process gives a good fit to the stochastically perturbed chemostats independent of the noise colour (see Supplementary Fig. 7 ). We estimated the density regulation parameter for the experimental runs in scenario 3 using the Matlab function ‘arcov’ and obtained a -values in the range 0.93–0.99, with a median of a =0.97. We used this value as our standard parameter (for example, in Fig. 3 ). With some algebra the correlation coefficient of the two AR(1) processes can be calculated as [21] , [55] Note that the synchrony amplification r p / r does not depend on the correlation of the generating noises ρ . The Moran theorem r p = r holds true only if the noise colours of both populations are identical α = β . Otherwise, for non-identical noise colours α ≠ β , the cross-correlation between the two independent populations will exceed the correlation of the environmental noises, r p > r (enhanced Moran effect). Note that our derivation of the synchrony amplification depends on a number of implicit assumptions about the ecological situation that we model in our system. In particular, the precise analytic form of equation (7) is limited to the case of linear population dynamics, identical populations and habitat properties, the absence of dispersal or other forms of population interactions, and the fact that the noises have been generated by an AR(1) process. See Supplementary Methods and Supplementary Figs 10–14 for different generalizations of this result, including different measures of cross-correlation, non-identical and density-dependent population dynamics, or long-term correlated noises. The dependence of the synchrony amplification factor r p / r on the noise colours and the density regulation parameter is visualized in Supplementary Figs 8 and 9 . In general, r p / r increases with the difference in noise colours between the two populations. For small differences in noise colours it is possible to simplify equation (7) by Taylor expansion. Setting ε= β − α we obtain which can be expanded for small values of a to yield (equation 1, main text). If the noise colour is restricted to red noise ( α , β ε[0,1]) the maximal amplification of synchrony in equation (7) is obtained as a function of r for while, as function of ε=| α − β |, the synchrony amplification is restricted in the range These ranges are indicated as black lines in Fig. 3a,b . Chemostat simulations In addition to the simulations with the more generic autoregressive models, we also used an ordinary differential equation model to provide a more specific simulation of the population dynamics in our experimental system. The model describes a chemostat, consisting of an algal population of density N that grows on nitrogen as an essential resource with concentration R [56] , [57] . The growth-limiting resource is supplied from an external medium with input concentration R i . The flow through the system is described by the time-dependent dilution rate δ ( t ). Resource uptake follows Monod kinetics f ( R )= u max R /( K + R ) with maximal growth rate u max and half-saturation constant K . The algae grow according to the absorbed amount of resource, f ( R ) N , and are washed out from the system by δ ( t ) N . To describe the stochastic forcing, the dilution rates were assumed to be time-dependent, δ ( t ), and were simulated as piecewise-constant stochastic function of time, where the dilution rate is adjusted to a new value at fixed time intervals (every or 1 or 2 h). Following the design of our experimental setting, we simulate two uncoupled chemostat systems where the time course of the dilution rates is cross-correlated by a pre-determined value, ρ , and, depending on the simulation run, may also be autocorrelated in time. Thereby, δ ( t ) is taken either to be identical to the time course of the dilution rates in the experimental runs ( Fig. 3 , main text) or, to obtain longer simulation runs, we generate correlated random numbers from the same statistical distributions as in the experiments. As shown in Supplementary Fig. 2 , the model is able to accurately describe the population dynamics in our laboratory experiment. Parameter values were chosen to resemble the experimental system. The resource concentration of the external supply medium R i and the average dilution rate ‹ δ › were chosen according to the values of the chemostat experiments. The parameter values for maximum growth rate, u max , and half-saturation constant, K , were chosen by hand to provide an optimal fit to our experimental results. We used the maximum growth rate u max =2.5 per day and the half-saturation constant K =45 μmol l −1 . These values are within the range of parameters that are reported for related green algae in the literature. For example, u max =0.79 per day ( Chlorella pyrenoidosa [58] ), u max =0.37–1.92 per day ( C. pyrenoidosa [59] ), K =0.89 μmol l −1 ( C. vulgaris [60] ), K =4.5 μmol l −1 ( C. pyrenoidosa [58] ) and K =230 μmol l −1 ( C. pyrenoidosa [61] ). The population synchrony, obtained from numerical simulations, was highly robust to changes in these model parameters. How to cite this article : Massie, T. M. et al . Enhanced Moran effect by spatial variation in environmental autocorrelation. Nat. Commun. 6:5993 doi: 10.1038/ncomms6993 (2015).